Deterministic and electrically tunable bright single-photon source The scalability of a quantum network based on semiconductor quantum dots lies in the possibility of having an electrical control of the quantum dot state as well as controlling its spontaneous emission. The technological challenge is then to define electrical contacts on photonic microstructures optimally coupled to a single quantum emitter. Here we present a novel photonic structure and a technology allowing the deterministic implementation of electrical control for a quantum dot in a microcavity. The device consists of a micropillar connected to a planar cavity through one-dimensional wires; confined optical modes are evidenced with quality factors as high as 33,000. We develop an advanced in-situ lithography technique and demonstrate the deterministic spatial and spectral coupling of a single quantum dot to the connected pillar cavity. Combining this cavity design and technology with a diode structure, we demonstrate a deterministic and electrically tunable single-photon source with an extraction efficiency of around 53±9%. In recent years, many key features have been demonstrated with semiconductor quantum dots (QDs) showing their potential for quantum information processing: ultrabright sources of single photons [1] , [2] or entangled photon pairs [3] , highly indistinguishable photons [4] , entangled light-emitting diodes [5] , single-spin optical manipulation [6] , long spin coherence time [7] , ultrafast optical gates at the few photon scales [8] , [9] , [10] and spin–photon entanglement [11] , [12] among others. To build a scalable solid-state quantum network, two tools have appeared essential to make these individual functionalities deterministic and efficient. First, one needs a control of the QD state to deterministically inject an electron or a hole spin in the QD [13] , to tune the QD resonance to a target wavelength [14] , to control the coupling of two coupled QDs [15] or to control the exciton fine structure splitting [16] . Inserting the QDs in doped structures and applying an electric field has been shown to be an efficient way to achieve this first requirement. Second, a highly efficient ‘single QD’–‘single photon’ interface is needed to ensure that every photon emitted by the QD is collected or, symmetrically, that every photon sent to control the QD state interacts with the QD. For this second requirement, an efficient way is to control the spontaneous emission of the QD using a microcavity [2] , [17] or a photonic nanowire [1] . Combining electrical control with an efficient ‘single photon’–‘single QD’ interface has appeared to be technologically challenging. The first difficulty lies in defining electrical contacts on structures presenting lateral sizes of a few hundred nanometres to a few microns like nanowires or microcavities [18] , [19] . So far, no electrical control has been demonstrated for bright QD single-photon sources based on nanowires and only one group has been able to apply an electric field on a micropillar cavity [19] , [20] , although with a highly challenging technology. An alternative approach has consisted of defining electrical contacts on large mesa structures and confining the optical field using lateral oxidation [21] . The cavity size is then controlled through a precise control of the oxidation process [22] . The second difficulty lies in the necessity to position the QD precisely in the photonic structure to ensure a good coupling between the QD and the optical mode [23] , [24] . Encouraging first results have recently been obtained with site-controlled QDs, yet without a control on the spectral matching of the QD and the cavity mode energies [25] . Overall, the state-of-the-art in terms of extraction efficiency for an electrically controlled single-photon source is 38%, obtained without a deterministic control of the QD-cavity coupling [20] , [21] . Here, we present a cavity design which allows confinement of the optical mode in the three spatial directions while preserving large structures to easily define electrical contacts. The cavity consists of a micropillar connected to a 25 × 25 μm 2 wide frame through one-dimensional wires, as illustrated in Fig. 1a . We show that high quality factors, up to 33,000, can be reached with connected pillar structures. We demonstrate the potential of this new cavity design by fabricating a tunable bright single-photon source through application of an electrical bias. Connected pillar structures are defined on a p-i-n doped planar cavity embedding a QD layer. An advanced in-situ lithography technique [24] is developed to deterministically couple a single QD to a connected pillar cavity. Fine tuning of the QD line into the cavity resonance is obtained through the confined Stark effect: at resonance, an extraction efficiency of 53±9% is estimated. 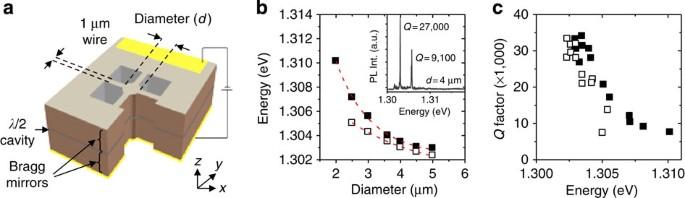Figure 1: Novel design for electrically connected micropillar cavities. (a) Schematic of the structure: a circular micropillar with diameterdis connected to a 25 × 25 μm2frame through four 1-μm wide one-dimensional wires. Electrical contacts are defined on the frame. In the following, a single quantum dot is inserted in the centre of the connected pillar. (b) Energy of the fundamental mode in isolated pillars (solid symbols) and connected pillars (open symbols). The dashed lines are guides to the eyes. Inset: photoluminescence (PL) spectrum of the connected pillar with a diameter of 4 μm. (c) Quality factor of the fundamental mode for the isolated (solid) and connected pillars (open). Figure 1: Novel design for electrically connected micropillar cavities. ( a ) Schematic of the structure: a circular micropillar with diameter d is connected to a 25 × 25 μm 2 frame through four 1-μm wide one-dimensional wires. Electrical contacts are defined on the frame. In the following, a single quantum dot is inserted in the centre of the connected pillar. ( b ) Energy of the fundamental mode in isolated pillars (solid symbols) and connected pillars (open symbols). The dashed lines are guides to the eyes. Inset: photoluminescence (PL) spectrum of the connected pillar with a diameter of 4 μm. ( c ) Quality factor of the fundamental mode for the isolated (solid) and connected pillars (open). Full size image Optical field confinement in connected pillars Micropillar cavities are few micron wide structures etched in a planar cavity. Lateral confinement of the optical field arises from the high refractive index contrast between the air and the semiconductor: for circular pillars, the transverse optical modes are essentially those of an optical fibre [17] . To allow the application of an electric field on such pillar cavities, we propose the connected pillar structure illustrated in Fig. 1a : a circular pillar with diameter d is connected to a 25 × 25 μm 2 frame through four 1 μm wide one-dimensional wires. The electrical contact will be defined on the frame. For isolated pillars with diameters larger than 1.5 μm, the optical field hardly penetrates the air for the first confined modes. We therefore expect the fundamental mode of the connected pillar cavity to be confined in the centre of the pillar with a low penetration into the one-dimensional wires. We study the confinement of the optical field in connected pillars and compare with the case of isolated pillars. To do so, a λ-GaAs cavity presenting a quality factor Q exceeding 35,000 is used in order to investigate the possibility of obtaining high quality factors with connected pillar structures. Both isolated and connected pillars cavities are fabricated from the same wafer (see Methods). The emission of a large QD density inserted in the cavity acts as a white light source and allows probing the cavity modes. The inset in Fig. 1b presents a typical spectrum measured on a connected pillar cavity with d =4 μm. Two discrete lines are visible corresponding to the fundamental and first confined optical modes. Figure 1b presents the measured energy of the fundamental mode for the connected and isolated pillar cavities as a function of the diameter. For a given diameter, the energy of the connected pillar is lower than that of the isolated one: field penetration in the wires results in a larger effective volume. Considering that in isolated pillars, the larger the diameter, the narrower is the mode radiation pattern [26] , this observation further means that connected pillar cavities present more directional radiation patterns than isolated ones with the same diameter. Figure 1c presents the measured quality factor for both types of pillar as a function of the mode energy so as to compare pillars presenting equivalent effective volumes. Connected pillars present slightly lower quality factors than isolated ones suggesting that additional in-plane leakage occurs due to guiding effect in the wires. However, very high quality factors are obtained on connected pillars, as high as 2 × 10 4 –2.5 × 10 4 for a mode volume corresponding to that of isolated pillars with 3–3.5 μm diameter. This shows that connected pillar cavities have good enough characteristics to reach the strong coupling regime with a single QD [27] . In the following, we demonstrate the potential of this cavity structure by deterministically coupling a single QD to a connected pillar cavity and fabricating an electrically tunable bright single-photon source. To do so, a planar cavity structure with a low quality factor Q 0 is used in order to minimize the detrimental effect of sidewall losses on the source brightness [2] . Advanced in-situ lithography technique Although single QDs have been shown to be good single-photon sources [28] , techniques are needed to efficiently collect their emission. Indeed, total internal reflection in the high refractive index semiconductor leads to collection efficiencies around a few percent for bulk structures. One way to solve this difficulty is to couple the QD to a confined cavity mode. Acceleration of spontaneous emission by the so called Purcell factor F P then ensures that a large fraction of the emitted photons are emitted in the cavity mode. For pillar cavities, since the spontaneous emission into leaky modes is hardly modified as compared with the case of bulk structures [29] , this fraction is given by β = (ref. 17 ). However, this requires that the QD is located at the maximum of the electric field of the confined mode and that the QD optical transition is spectrally resonant to the cavity mode. In 2008, we proposed a technique to achieve this deterministic coupling for QD in pillar cavities [24] . A planar cavity structure embedding a dilute layer of randomly distributed QDs is spin coated with a positive photoresist. The sample is brought at low temperature to measure the QD emission. An 850-nm laser line exciting the QD emission without exposing the resist allows measuring the QD position with a 50-nm accuracy through mapping its emission intensity. A second 532-nm laser line is then used to expose a disk centred on the QD with a diameter adjusted for the pillar fundamental mode to match the QD spectral resonance. Here, an advanced in-situ lithography technique is developped to allow the deterministic insertion of a single QD in a connected pillar cavity. The setup is based on a three colour attoCFM1 attocube confocal microscope. An optical microscopy insert is cooled down to 4.2 K using a helium bath cryostat providing long term stability. Three fibre-based optical lines (two for laser excitation at 850 nm and 532 nm, one for QD emission collection) are collimated and sent in free space down the insert onto a microscope objective with NA 0.75. The sample is placed on a piezo-actuators stack in the focal plane of the microscope objective as schematically described in Fig. 2a . An alignment step allows superimposing the laser excitation lines with a 50-nm accuracy by monitoring the reflected signal from each laser line while scanning the lasers on a metallic grating. Capacitive sensors located on the piezo-actuators stack allow a reading of the sample absolute position with an accuracy greater than 10 nm. This absolute control of the sample position, an electronically controlled shutter on the green laser line and a custom developed software allow writing sophisticated patterns in the resist centred on a selected single QD. 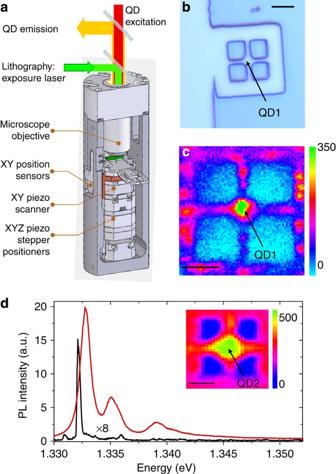Figure 2: Technology developed to align a connected pillar on a single quantum dot. (a) Schematic illustration of thein-situsetup used for writing sophisticated patterns centred on a single QD. (b) Optical image of an in-situ lithography pattern defined in the photoresist and centred on a single QD. Scale bar, 10 μm. (c) Emission intensity map selecting a 5-nm wavelength range around the fundamental mode of the connected pillar. Scale bar, 5 μm. (d) PL spectrum measured on a second connected pillar device, at high excitation power (red) or low excitation power (black). Inset: emission intensity map. Scale bar, 3 μm. Figure 2b presents an optical microscope image of a connected pillar shape defined in the photoresist by in-situ lithography at 4.2 K, obtained after developing the resist. Subsequent steps involve metal deposition, lift-off and semiconductor etching to obtain the connected pillar device [24] . Figure 2c shows a mapping of the emission intensity obtained on the etched structure measured in the same confocal setup. We detect the emission intensity spectrally filtered in a 5-nm wide wavelength range around the fundamental mode of the connected pillar, while scanning the sample with respect to the excitation laser beam. Bright spots are visible on the right part of the image in the frame area of the device: these spots arise from other QDs emitting in this wavelength range in the planar cavity structure. A much stronger signal arises from the QD centred in the pillar structure, first indication of a higher extraction efficiency provided by the Purcell effect. Figure 2d shows an emission spectrum recorded on another device (coupled to QD2) for excitation centred on the pillar (inset shows the emission mapping when selecting the fundamental mode spectral range). At high excitation power, three confined modes of the structure are observed. At low excitation power, a single QD emission line, spectrally well matched to the connected pillar fundamental mode is observed. Figure 2: Technology developed to align a connected pillar on a single quantum dot. ( a ) Schematic illustration of the in-situ setup used for writing sophisticated patterns centred on a single QD. ( b ) Optical image of an in-situ lithography pattern defined in the photoresist and centred on a single QD. Scale bar, 10 μm. ( c ) Emission intensity map selecting a 5-nm wavelength range around the fundamental mode of the connected pillar. Scale bar, 5 μm. ( d ) PL spectrum measured on a second connected pillar device, at high excitation power (red) or low excitation power (black). Inset: emission intensity map. Scale bar, 3 μm. Full size image Electrical tunability of the source In order to apply an electric field and finely tune the QD emission energy, the above technology was performed on a planar cavity embedding a diode structure (see Methods). The QD layer is centred in a 40-nm wide GaAs layer embedded in an undoped antiguiding λ /2 AlAs cavity [14] . As shown in Fig. 3a , the top (bottom) Bragg mirror with 16 (36) pairs is gradually p-doped (n-doped). When performing the in-situ lithography step as well as for the measurements presented in Fig. 2c,d , the structure is not electrically connected and no voltage is applied. Non-resonant optical excitation of carriers allows flattening the bands around the QD layer and observing QD emission. The 25 × 25 μm 2 frame surrounding the connected pillars are defined so as to overlap 100 × 100 μm 2 frames, on which metallic deposition and bonding is realized to define the top p-contact (see Fig. 3b ). Standard n-contact is defined on the back of the sample. In the following, the device is optically excited with a continuous wave laser at 850 nm. 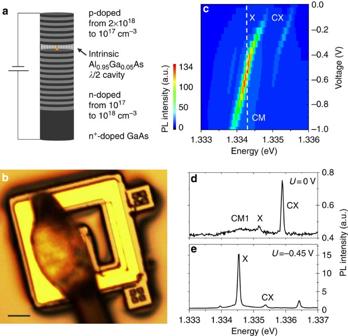Figure 3: Electrically tunable single-photon source. (a) Schematic sample structure with doping configuration. (b) Optical photograph of the bonded sample: two connected pillar devices are visible on the right side. During the in-situ lithography, we made sure that frame of the connected pillar overlaps a large frame where bonding is realized. Scale bar, 25 μm. (c) Emission intensity as a function of energy and applied electric field recorded at 35 K. (d,e) PL spectra measured for 0 V (d) and −0.45 V (e). Figure 3d shows the emission spectrum obtained for the device embedding QD1 at zero bias U =0 for a temperature of 35 K. The charge exciton (CX) and the neutral exciton (X) of QD1 are slightly detuned on the high energy side of the pillar fundamental mode (CM1). By application of a negative voltage, the QD emission lines shift towards lower energy and the X line is tuned throughout the mode resonance as evidenced in Fig. 3c , showing the emission intensity map as a function of energy and applied voltage. For a voltage U =−0.45 V ( Fig. 3e ), the QD1 X line is resonant to the cavity mode: a strong increase of the emission intensity is observed. This strong increase is partially due to Purcell effect as we show hereafter. Yet, carrier capture processes into the QD also vary with the applied voltage: similar measurements on QDs in the planar cavity of the frame show that the QD energy can be tuned over 1.4 meV for 0> U >−1 V. For higher negative voltage, the carriers created in the QD efficiently tunnel into the GaAs barriers and the QD emission vanishes. Note that the exciton of QD1 presents a positive detuning of 1.5 meV at 4 K and U =0. The electrical tuning range demonstrated above is almost enough to bring the exciton line in resonance, but not to tune the exciton throughout the mode. To do so, here we operate the device at 35 K. Figure 3: Electrically tunable single-photon source. ( a ) Schematic sample structure with doping configuration. ( b ) Optical photograph of the bonded sample: two connected pillar devices are visible on the right side. During the in-situ lithography, we made sure that frame of the connected pillar overlaps a large frame where bonding is realized. Scale bar, 25 μm. ( c ) Emission intensity as a function of energy and applied electric field recorded at 35 K. ( d , e ) PL spectra measured for 0 V ( d ) and −0.45 V ( e ). Full size image Single-photon emission and Purcell effect We now study the emission dynamics and photon statistics of the source. 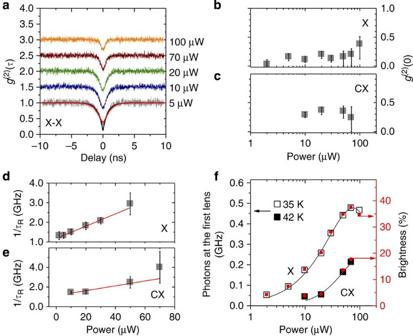Figure 4: Source characteristics. Photon statistics, Purcell effect and brightness. (a) Second order autocorrelation functiong(2)(τ) measured for X tuned into resonance with cavity mode CM1. Plots are vertically shifted for clarity. Red (black) line is a fit to the data obtained at 5 μW, convoluted (deconvoluted) with the setup temporal response. (b,c). Measuredg(2)(0) for the X and CX lines as a function of power. The values are corrected from the setup time resolution (see Methods). (d,e) Inverse of the correlation rise time as a function of power for X (T=35 K) and CX (T=42 K) forU=−0.45 V. The error bars are calculated taking into account the detector jitter time (see Methods). Red lines are linear fit to the experimental data using+gwheregis proportional to the excitation power. (f) Left axis: power dependence of the single-photon rate collected in the first lens for the X line (35 K, open black symbols) and the CX line (42 K, solid black symbols). The lines are theoretical fits∝(P/Psat)xwherePis the excitation power andPsatthe saturation power for the transition.x=0.9 for the X line andx=1.5 for the CX line. Right axis, red circular symbols: Brightness as a function of the excitation power. CX, charged exciton; X, neutral exciton. Figure 4a presents the autocorrelation function measured on the X line tuned into resonance with the cavity mode ( U =−0.45 V) for different excitation powers. Figure 4b presents the autocorrelation function at zero delay g (2) (0) extracted from the measurements and corrected from the setup temporal resolution, as explained in the Methods section. A good single-photon purity with g (2) (0)<0.2 is obtained up to saturation. From the experimental curves presented in Fig. 4a , we can also extract the deconvoluted rise time τ R of the autocorrelation function as a function of the excitation power. This rise time τ R is related to the X radiative lifetime τ X through + g where g is the pumping rate [30] . Figure 4d presents as a function of power, showing the expected linear dependence. For g =0 we find τ X =0.82±0.03 ns. Performing similar measurements for several reference QDs in the planar cavity for the same applied voltage, we find an average X lifetime of =1.45±0.1 ns. From this measurement, we deduce a Purcell factor of F P = −1=0.8±0.08. This measured value is close to the expected Purcell factor =1.1 calculated considering that Q =1300 for the mode and that this connected pillar presents the same effective volume as an isolated pillar with diameter 4.1 μm, as estimated considering the fundamental mode energy. Figure 4: Source characteristics. Photon statistics, Purcell effect and brightness. ( a ) Second order autocorrelation function g (2) ( τ ) measured for X tuned into resonance with cavity mode CM1. Plots are vertically shifted for clarity. Red (black) line is a fit to the data obtained at 5 μW, convoluted (deconvoluted) with the setup temporal response. ( b , c ). Measured g (2) (0) for the X and CX lines as a function of power. The values are corrected from the setup time resolution (see Methods). ( d , e ) Inverse of the correlation rise time as a function of power for X ( T =35 K) and CX ( T =42 K) for U =−0.45 V. The error bars are calculated taking into account the detector jitter time (see Methods). Red lines are linear fit to the experimental data using + g where g is proportional to the excitation power. ( f ) Left axis: power dependence of the single-photon rate collected in the first lens for the X line (35 K, open black symbols) and the CX line (42 K, solid black symbols). The lines are theoretical fits ∝ ( P / P sat ) x where P is the excitation power and P sat the saturation power for the transition. x =0.9 for the X line and x =1.5 for the CX line. Right axis, red circular symbols: Brightness as a function of the excitation power. CX, charged exciton; X, neutral exciton. Full size image Brightness and extraction efficiency Finally, we evaluate the brightness as well as the extraction efficiency of the device. For these measurements, the source emission is collected using a microscope objective with a 0.4 numerical aperture, sufficient to collect the mode full radiation pattern [26] . Figure 4f shows the photon count rate for the X line I X measured on the detector as a function of excitation power, reaching values as high as 4.08±0.002 MHz at saturation. The detection efficiency of the whole setup has been measured to be =0.0084±0.0008 in the present experimental conditions, leading to a photon rate collected in the first lens of I X / =0.48±0.05 GHz. Under continuous wave excitation, the photon rate is inversely proportional to the radiative lifetime of the transition. As a result, the source brightness, defined as the number of photons collected per excitation cycle of the QD is given by , where the square root allows correcting from multiphoton emission [31] . As shown on the right scale of Fig. 4f , a source brightness of 37±7% collected photon per cycle is demonstrated for the X line. The brightness of the source is the product of the extraction efficiency with the occupation factor p X of the QD X state. In the present measurement, the QD is found to be either in the neutral exciton X state or in the charged exciton state CX. To determine the respective occupation factors p X and p CX , we keep the voltage constant and increase the temperature from 35–42 K to bring the CX in resonance into the cavity mode. Given the small temperature change, we assume that capture processes are mostly unchanged. g (2) (0) measurements allow measuring a radiative decay time of τ CX =0.88±0.16 ns (see Fig. 4e ). The intensity of the CX line as a function of power ( Fig. 4f ) shows brightness at saturation of 17±6%. From this we deduce p X =0.69 and p CX =0.31 and estimate the extraction efficiency to be around 53±9% in a 0.4 numerical aperture. Knowing the cavity characteristics, the expected device extraction efficiency is given by . With Q ≈ Q 0 and =1.1, the expected extraction efficiency is around 52%, very close to the experimental one. We have demonstrated that by connecting pillars to a larger frame, one can both control the spontaneous emission of a single QD and apply an electric field on the structure. The extraction efficiency of 53±9% as well as brightness of 37±7% constitute state of the art results for electrically controlled sources [20] , [21] . They are obtained here with a fully deterministic technique, relying on an advanced in-situ lithography technique. The electrical tuning range of 1.4 meV reported here is limited by the thick GaAs barriers around the QD layer. Thinner barriers have previously been used to greatly increase this tuning range without significant reduction of the oscillator strength [14] . To fabricate several bright single-photon sources with the exact same emission wavelength, connected pillars with the same diameters can be centred on single QDs using in-situ lithography. The QD resonance would be chosen during the lithography to be slightly detuned on the high energy side of the mode so that it can be brought in resonance through the Stark effect. The use of a low quality factor mode for the cavity further allows the very fine tuning of two QD sources, without any loss in terms of brightness. Note that the demonstrated extraction efficiency is limited here by the low quality factor of the planar cavity and large volume of the connected pillar under study. Smaller connected pillar diameters or larger planar cavity quality factors should allow reaching state-of-the-art extraction efficiencies like in isolated pillars [2] . We expect that the in-situ lithography process can further be improved to minimize the wire width to 500 nm and further reduce the mode volume. Nevertheless, our work shows that, with the current state of the technology, the proposed cavity design is ready to be used to reach the strong coupling regime. Finally, with a proper optimizing of the doping in the structure to minimize absorption losses, the same technology should allow controlling the charge state of a single QD in a cavity. This would constitute an important step towards a deterministic spin–photon interface, a building block for a scalable solid-state quantum network [32] , [33] , [34] . Diode structure Two samples grown by molecular beam epitaxy are studied in the present work. The first one is used to study the properties of the optical modes in connected pillar structures ( Fig. 1 ). It is an undoped sample, consisting a λ cavity sandwiched within two Bragg mirrors with 30 pairs of alternating Al 0.95 Ga 0.05 As/GaAs λ /4 thick layers. The cavity embeds a QD layer with high spatial and spectral density. The quality factor of the planar cavity exceeds 35,000. To fabricate the pillars and isolated pillars, a standard e-beam lithography is used. The second one is a doped cavity structure used to fabricate the electrically tunable single-photon source ( Figs 2 , 3 , 4 ). A spatially diluted QD layer is embedded in a 40-nm wide GaAs layer centred in an undoped antiguiding λ /2 AlAs cavity [14] . The top (bottom) Bragg mirror with 16 (36) pairs is gradually p-doped (n-doped). The quality factor of the planar cavity mode is around 1,300. We minimize the losses induced by the doping on the cavity mode by gradually doping the Bragg mirrors. The Si n-doping changes gradually from 2 × 10 18 cm −3 to 1 × 10 17 cm −3 from the bottom-mirrors towards the undoped cavity. Symmetrically, the C p-doping increases progressively from 1 × 10 17 cm −3 to 1 × 10 18 cm −3 towards the top-mirrors. After resist deposition, a standard optical lithography is performed to define the 100 × 100 μm 2 frame. The low temperature in-situ lithography, as described in the text, is then used to define the cavities centred on selected QDs. We make sure that the 25 × 25 μm 2 frame overlaps with the larger ones. After pillar etching, the top p-contacts is defined on the large frame using a second standard optical lithography step, Ti/Au deposition and lift-off. All the devices have the same ground: Ni/Ge/Au/Ni/Au n-contact on the bottom n + -GaAs substrate. Optical measurements All measurements are performed with a continuous wave 850-nm excitation laser. To characterize the source, the device is placed in a helium flow cryostat and the QD emission is collected through a microscope objective with 0.4 numerical aperture. The emission is sent to a Hanbury Brown and Twiss setup consisting of a 50/50 beam splitter, sending the emission towards two spectrometers coupled to coupled charged devices or single-photon avalanche photodiodes. To measure the extraction efficiency of the source, all optical elements of the detection path have been calibrated using a continuous wave laser at 930 nm. The transmission of the spectrometer and the detection efficiency of the single-photon avalanche photodiodes are estimated by measuring a pulsed laser signal of known power for which we can deduce the number of incident photons per pulse. Data analysis for lifetime measurements The time resolution of a single detector (including the detector jitter and the time response of the electronics ) is determined measuring the response of the system to a picosecond laser pulse. This measured response function is fitted using a symmetric exponential decay function f ( t )= with τ setup =350±17 ps. We fit the measured correlation curves using the convolution of the theoretical function g (2) ( t )=1−(1− g (2) (0)) with f (ref. 35 ) and extract the deconvoluted values for the autocorrelation function at zero delay g (2) (0) and the rise time τ R with an error bar Δ . The experimental error on the detector time resolution Δ τ setup =35 ps leads to an additional error Δ on the extracted τ R so that the total error bar is Δ τ R =Δ +Δ . Since the deconvoluted τ R is very close to the one obtained using the sum of the square approximation τ R ≈ where τ exp is the rise time obtained by fitting the experimental data directly with g (2) ( t ) =1−(1− (0)) , we estimate that Δ ≈Δ τ setup τ setup . We find that the error bars on the rise time τ R are between 10 and 20% for the exciton line and between 8 and 40% for the charged exciton. The largest error bars are obtained at low power because of lower signal-to-noise ratio (large Δ ) and at high power because the rise time gets closer to τ setup (large Δ ). Because 1/ τ R =1/ τ + g where τ is the lifetime of the line and g is proportional to the pumping rate, a linear fit of the measured 1/ τ R as a function of power allows extracting τ . As can be seen in Fig. 4d , the experimental points for 1/ τ R for the exciton are very well aligned: the fitting linear procedure results in a exciton lifetime of 820±30 ps. Note that the fitting procedure takes into account the total experimental errors on τ R . For the charged exciton, larger error bars on τ R result in a larger error bar (20%) on the trion lifetime: we find 0.88±0.16 ns. How to cite this article: Nowak, A. K. et al . Deterministic and electrically tunable bright single-photon source. Nat. Commun. 5:3240 doi: 10.1038/ncomms4240 (2014).